Glycogen shortage during fasting triggers liver–brain–adipose neurocircuitry to facilitate fat utilization During fasting, animals maintain their energy balance by shifting their energy source from carbohydrates to triglycerides. However, the trigger for this switch has not yet been entirely elucidated. Here we show that a selective hepatic vagotomy slows the speed of fat consumption by attenuating sympathetic nerve-mediated lipolysis in adipose tissue. Hepatic glycogen pre-loading by the adenoviral overexpression of glycogen synthase or the transcription factor TFE3 abolished this liver–brain–adipose axis activation. Moreover, the blockade of glycogenolysis through the knockdown of the glycogen phosphorylase gene and the resulting elevation in the glycogen content abolished the lipolytic signal from the liver, indicating that glycogen is the key to triggering this neurocircuitry. These results demonstrate that liver glycogen shortage activates a liver–brain–adipose neural axis that has an important role in switching the fuel source from glycogen to triglycerides under prolonged fasting conditions. A sufficient energy supply is essential for life; consequently, multiple mechanisms have evolved to ensure both energy availability and conservation during fasting. During fasting, liver glycogen, a glucose-storage polymer, is initially mobilized to replenish blood glucose (glycogenolysis). Major changes in metabolism are known to occur as the glycogen supply dwindles; when glycogen storage in the liver is depleted, stored adipose tissue triglycerides are released into the circulation as fatty acids and glycerol. The released fatty acids are directly oxidized as an energy source by some tissues (liver and muscle), or are metabolized by the liver to ketone bodies for use by tissues, notably the brain that cannot utilize fatty acids, while the glycerol is converted by the liver into glucose (gluconeogenesis). Among the mechanisms that prompt this shift in energy source from liver glycogen to adipose triglycerides are changes in blood hormones; when an animal is fasting, the body senses a drop in the glucose concentration at sites such as the pancreatic islets and brain and responds by reducing insulin secretion from islet β cells and by increasing glucagon secretion from islet α cells. Another response is sympathetic adrenal stimulation causing increased epinephrine levels [1] . However, whether the trigger that switches the major energy source from hepatic glycogen to adipose tissue triglycerides is comprised only of the drop in blood glucose level and the concomitant changes in metabolic hormone levels has not yet been determined. Here we show that liver glycogen shortage directly activates a liver–brain–adipose neural axis independently of blood glucose and insulin/glucagon levels, having an important role in switching the fuel source from glycogen to triglycerides under prolonged fasting conditions ( Supplementary Fig. S1 ). Selective hepatic vagotomy preserves fasting fat pad mass To examine the role of the hepato-vagal nerve pathway in the regulation of lipolysis in adipose tissue, we dissected the hepatic branch of the vagus nerve and observed the metabolic changes in epididymal fat pads during fasting. Three weeks after a selective hepatic vagotomy (HVx) was performed using microsurgery, once the animals had recovered their body weight and their food intake had returned to normal [2] ( Supplementary Fig. S2a,b ), the mice were killed in a fasting state. As shown in Fig. 1a–e , the vagotomized mice fasted for 24 h lost significantly less fat and displayed larger adipocytes than mice with a sham surgery (isolation of the nerve without resection). The same effect as that seen after the HVx was also observed after capsaicin treatment, which chemically ablates only the afferent vagus nerve composed of unmyelinated fibres ( Fig. 1a–e , Supplementary Fig. S3a,b ). This effect of HVx or capsaicin treatment was not seen in subcutaneous fat ( Fig. 1e ). 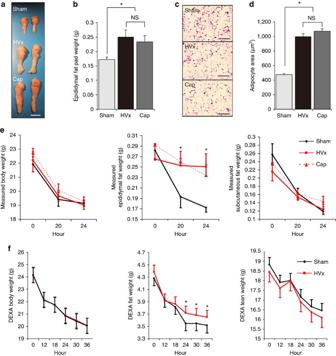Figure 1: Selective HVx preserves fasting fat pad mass. (a) Gross appearance of epididymal fat in sham, hepatic vagotomized (HVx) and capsaicin-treated (Cap) mice. (b) Weight of remnant epididymal fat tissue in sham, HVx and Cap model after 24 h of fasting. Scale bar, 5 mm. (n=7). (c) Microscopic appearance of HE-stained epididymal fat tissue. Scale bar, 100 μm. (d) Morphometry of adipocytes in sham, HVx and Cap animals. (n=3, 10 fields per a section). (e) Total body weight, weight of epididymal fat pad and subcutaneous fat in 0, 20 and 24 h fasting mice. (n=5–7). (f) Changes in body weight (left), fat weight (middle) and lean body weight (right) during fasting measured using DEXA. (n=4–7). *P<0.05 versus sham group (by Tukey’spost-hoctest). Error bars, s.e.m. Figure 1f shows that the body fat weight loss during fasting was significantly retarded in HVx mice after 24 h when analysed using DEXA (digital energy X-ray analysis), while the total body weight in both the sham and HVx groups decreased similarly. Figure 1: Selective HVx preserves fasting fat pad mass. ( a ) Gross appearance of epididymal fat in sham, hepatic vagotomized (HVx) and capsaicin-treated (Cap) mice. ( b ) Weight of remnant epididymal fat tissue in sham, HVx and Cap model after 24 h of fasting. Scale bar, 5 mm. ( n =7). ( c ) Microscopic appearance of HE-stained epididymal fat tissue. Scale bar, 100 μm. ( d ) Morphometry of adipocytes in sham, HVx and Cap animals. ( n =3, 10 fields per a section). ( e ) Total body weight, weight of epididymal fat pad and subcutaneous fat in 0, 20 and 24 h fasting mice. ( n =5–7). ( f ) Changes in body weight (left), fat weight (middle) and lean body weight (right) during fasting measured using DEXA. ( n =4–7). * P <0.05 versus sham group (by Tukey’s post-hoc test). Error bars, s.e.m. Full size image Vagotomy suppresses sympathetic nerve-mediated lipolysis Next, we examined the metabolic changes in adipose tissue caused by HVx. When cAMP signalling, which is the second messenger mediating the lipolytic signal, was visualized using adenovirally delivered luciferase reporter driven by the cAMP response element (CRE-luc) using an in vivo imaging system, cAMP signalling in the epididymal fat was reduced by HVx ( Fig. 2a ). Accordingly, the activated form of hormone-sensitive lipase (HSL), phosphorylated at Ser 563, tended to be reduced by hepatic vagus nerve interference ( Fig. 2b ; Supplementary Fig. S4a ). The mRNA levels of HSL and adipose triglyceride lipase (ATGL) as well as pyruvate dehydrogenase kinase 4, a key enzyme regulating glyceroneogenesis that is induced by fasting or epinephrine treatment [3] , were also downregulated ( Fig. 2c ). There were no differences between HVx and capsaicin-treated groups, indicating that afferent signal is of key importance. These changes in lipolytic activities resulted in lower levels of plasma non-esterified fatty acids and glycerol in the HVx groups ( Fig. 2d ), leading to higher respiratory quotient and lower fat utilization per body despite the equal energy consumption ( Fig. 2e,f ). These differences were cancelled by guanethidine administration, which reduces the release of catecholamines from sympathetic nerves ( Fig. 2g , Supplementary Fig. S5a,b ) [4] . The plasma glucose, insulin, glucagon, catecholamines and FGF21 concentrations during fasting were not significantly different between the HVx and sham groups ( Fig. 2d , Supplementary Figs S6 and S7a,b ). These data demonstrate that the hepatic vagal signals control the lipolytic activities in adipose tissues through the sympathetic nervous system. 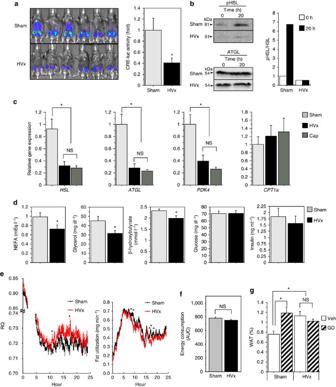Figure 2: Vagotomy suppresses sympathetic nerve-mediated lipolysis. (a),Ad-CRE-luc activities in adipose tissue visualized using IVIS Imaging System after 20 h of fasting. *P<0.05 versus sham group (by Student’st-test) (n=6). (b) Left, protein expressions assessed by western blot analysis using specific antibodies for Ser 563 phospho-HSL (p-HSL) and ATGL in epididymal adipose tissue of sham and HVx mice after 0 and 20 h of fasting. Right, quantification of the blot (ratio of p-HSL to total HSL) (n=5 pooled). (c) mRNA expressions in epididymal fat of 24 h fasting animals, examined by real-time quantitative PCR (RT–qPCR). *P<0.05 versus sham group (by Tukey’spost-hoctest) (n=7). (d) Circulating non-esterified fatty acid (NEFA), glycerol, β-hydroxybutyrate, glucose and insulin levels after 20 h of fasting. *P<0.05 versus sham group (by Student’st-test) (n=4–9). (e,f) Respiratory quotient (RQ), fat utilization and energy consumption measured using a calorimetric system. *P<0.05 versus sham group (by Student’st-test) (n=15–18). (g) Weight of remnant epididymal fat tissue in sham or HVx mice with or without guanethidine (GD) treatment after 24 h fasting. *P<0.05 versus sham group (by Tukey’spost-hoctest) (n=6–10). NS, not significant. Error bars, s.e.m. Figure 2: Vagotomy suppresses sympathetic nerve-mediated lipolysis. ( a ),Ad-CRE-luc activities in adipose tissue visualized using IVIS Imaging System after 20 h of fasting. * P <0.05 versus sham group (by Student’s t -test) ( n =6). ( b ) Left, protein expressions assessed by western blot analysis using specific antibodies for Ser 563 phospho-HSL (p-HSL) and ATGL in epididymal adipose tissue of sham and HVx mice after 0 and 20 h of fasting. Right, quantification of the blot (ratio of p-HSL to total HSL) ( n =5 pooled). ( c ) mRNA expressions in epididymal fat of 24 h fasting animals, examined by real-time quantitative PCR (RT–qPCR). * P <0.05 versus sham group (by Tukey’s post-hoc test) ( n =7). ( d ) Circulating non-esterified fatty acid (NEFA), glycerol, β-hydroxybutyrate, glucose and insulin levels after 20 h of fasting. * P <0.05 versus sham group (by Student’s t -test) ( n =4–9). ( e , f ) Respiratory quotient (RQ), fat utilization and energy consumption measured using a calorimetric system. * P <0.05 versus sham group (by Student’s t -test) ( n =15–18). ( g ) Weight of remnant epididymal fat tissue in sham or HVx mice with or without guanethidine (GD) treatment after 24 h fasting. * P <0.05 versus sham group (by Tukey’s post-hoc test) ( n =6–10). NS, not significant. Error bars, s.e.m. Full size image Glycogen loading cancels liver–brain–adipose axis activation Next, we explored the mechanism by which the liver–brain–adipose neurocircuitry is activated during fasting. First, the effect of the forced pre-loading of glycogen was tested; when glycogen synthase 2 ( Gys2 ) or the transcription factor TFE3, which promotes glycogen synthesis [5] , was overexpressed by adenoviral gene delivery to the liver, the hepatic glycogen contents and consequently the adipose tissue mass increased to the levels of those seen in vagotomized mice ( Fig. 3a,b,e,f , Supplementary Fig. S8a,b ). Consistent with this finding, the expressions of the lipolytic enzymes HSL and ATGL as well as the phosphorylated HSL levels were suppressed by Gys2 or TFE3 overexpression in the liver ( Fig. 3c,d,g,h ; Supplementary Fig. S4b,c ). These data indicate that hepatic glycogen loading abolishes the activation of the liver–brain–adipose axis during fasting. 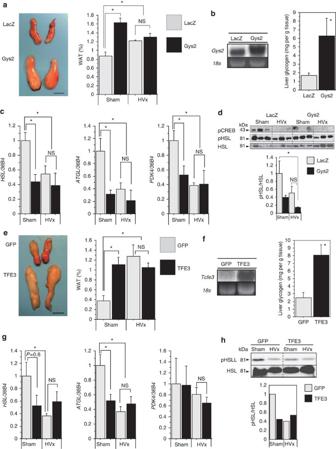Figure 3: Hepatic glycogen loading cancels liver–brain–adipose axis activation. (a,e) Gross appearance and weight of epididymal fat in Ad-CMV-Gys2 (a) or Ad-CMV-TFE3 (e) injected mice (filled bars) compared with control (grey bars; Ad-CMV-LacZ/GFP). Scale bar, 5 mm. *P<0.05 versus Ad-CMV-LacZ/GFP-treated sham group (by Tukey’spost-hoctest) (n=5–9). (b,f) Northern blots verifyingGys2orTFE3overexpression (three individual liver RNA samples pooled) and hepatic glycogen content in mice infected with Ad-CMV-Gys2 or Ad-CMV-TFE3. *P<0.05 versus Ad-CMV-LacZ/GFP-treated group (by Student’st-test) (n=5–14). (c,g) RT–qPCR analyses of HSL, ATGL and pyruvate dehydrogenase kinase 4 (PDK4) mRNA expression of epididymal fat inGys2- orTFE3-overexpressing mice in starvation. *P<0.05 versus Ad-CMV-LacZ/GFP-treated sham group (by Tukey’spost-hoctest) (n=4–9). (d,h) Protein expression of Ser 563 p-HSL and total HSL in epididymal adipose tissue ofGys2- orTFE3-overexpressing mice. (n=3 or three individual protein samples pooled). All mice are analysed on 24-h fasting condition. *P<0.05 versus Ad-CMV-LacZ-treated sham group (by Tukey's post-hoc test). NS, not significant. Error bars, s.e.m. Figure 3: Hepatic glycogen loading cancels liver–brain–adipose axis activation. ( a , e ) Gross appearance and weight of epididymal fat in Ad-CMV-Gys2 ( a ) or Ad-CMV-TFE3 ( e ) injected mice (filled bars) compared with control (grey bars; Ad-CMV-LacZ/GFP). Scale bar, 5 mm. * P <0.05 versus Ad-CMV-LacZ/GFP-treated sham group (by Tukey’s post-hoc test) ( n =5–9). ( b , f ) Northern blots verifying Gys2 or TFE3 overexpression (three individual liver RNA samples pooled) and hepatic glycogen content in mice infected with Ad-CMV-Gys2 or Ad-CMV-TFE3. * P <0.05 versus Ad-CMV-LacZ/GFP-treated group (by Student’s t -test) ( n =5–14). ( c , g ) RT–qPCR analyses of HSL, ATGL and pyruvate dehydrogenase kinase 4 (PDK4) mRNA expression of epididymal fat in Gys2 - or TFE3 -overexpressing mice in starvation. * P <0.05 versus Ad-CMV-LacZ/GFP-treated sham group (by Tukey’s post-hoc test) ( n =4–9). ( d , h ) Protein expression of Ser 563 p-HSL and total HSL in epididymal adipose tissue of Gys2 - or TFE3 -overexpressing mice. ( n =3 or three individual protein samples pooled). All mice are analysed on 24-h fasting condition. * P <0.05 versus Ad-CMV-LacZ-treated sham group (by Tukey's post-hoc test). NS, not significant. Error bars, s.e.m. Full size image Glycogenolysis blockade abolishes lipolytic signal from liver Conversely, when Gys2 expression was knocked down by adenovirally transferred short hairpin RNA (shRNA), and liver glycogen shortage was concomitantly exacerbated, the adipose tissue tended to shrink faster, and this tendency was cancelled by the HVx ( Fig. 4a,c–e , Supplementary Fig. S4d , Supplementary Table S1 ). Next, to distinguish which of the parameters, glycogen itself or its downstream metabolites, is the key to triggering liver–brain–adipose axis activation when depleted, the glycogen phosphorylase liver type gene ( Pygl ) was knocked down using shRNA ( Fig. 4b–e , Supplementary Fig. S4d , Supplementary Table S1 ); when glycogenolysis was suppressed by this RNA interference, the liver glycogen content was elevated and this in turn led to a decrease in lipolysis in the adipose tissue. This result demonstrates that the shortage of glycogen, but not that of the downstream metabolites, is the key to triggering the neurocircuitry. Meanwhile, AMP-activated kinases (AMPKs) were prone to be activated by the knockdown of glycogen phosphorylase ( Fig. 4f,g , Supplementary Fig. S4e ). 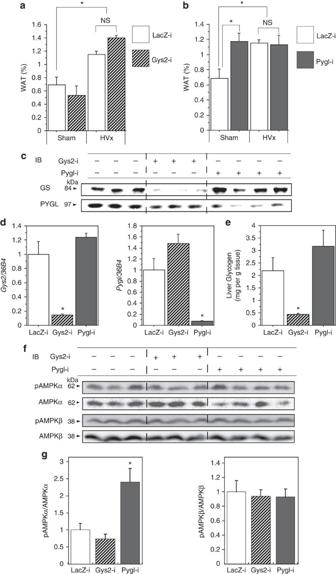Figure 4: Glycogenolysis blockade abolishes lipolytic signal from liver. (a,b) Weight of epididymal fat pad after fasting. Effects of short hairpin RNA expression adenovirus vector targeted forGys2(hatched bar,a) orPygl(filled bar,b). (n=4–8). (c) Immunoblot analysis of glycogen synthase (GS) and glycogen phosphorylase (PYGL) expression in the livers of Ad-Gys2-i or Ad-Pygl-i injected mice. (n=3–4). (d) RT–qPCR analysis of mRNA expression of glycogen synthase (Gys2) and glycogen phosphorylase (Pygl) genes. (n=3). (e) Liver glycogen content of mice infected with adenovirus expressing short hairpin RNA targeted forLacZ, Gys2orPygl(Ad-LacZ-i, Ad-Gys2-i or Ad-Pygl-I, respectively) (n=3–4). (f) Immunoblot analysis of Ser485-phosphorylated AMPKα (pAMPKα), total AMPKα, Ser181-phosphorylated AMPKβ (pAMPKβ) and total AMPKβ. Whole-cell lysates from the livers of mice infected with adenovirus expressing short hairpin RNA targeted forLacZ,Gys2orPygl(Ad-LacZ-i, Ad-Gys2-i or Ad-Pygl-i). (g) Quantified results of the data shown in (f), shown as the ratio of pAMPKα to total AMPKα and pAMPKβ to total AMPKβ. (n=3–4). All mice are analysed on 24-h fasting condition. *P<0.05 versus Ad-LacZ-i sham group (by Tukey’spost-hoctest). NS, not significant. Error bars, s.e.m. Figure 4: Glycogenolysis blockade abolishes lipolytic signal from liver. ( a , b ) Weight of epididymal fat pad after fasting. Effects of short hairpin RNA expression adenovirus vector targeted for Gys2 (hatched bar, a ) or Pygl (filled bar, b ). ( n =4–8). ( c ) Immunoblot analysis of glycogen synthase (GS) and glycogen phosphorylase (PYGL) expression in the livers of Ad-Gys2-i or Ad-Pygl-i injected mice. ( n =3–4). ( d ) RT–qPCR analysis of mRNA expression of glycogen synthase ( Gys2 ) and glycogen phosphorylase ( Pygl ) genes. ( n =3). ( e ) Liver glycogen content of mice infected with adenovirus expressing short hairpin RNA targeted for LacZ, Gys2 or Pygl (Ad-LacZ-i, Ad-Gys2-i or Ad-Pygl-I, respectively) ( n =3–4). ( f ) Immunoblot analysis of Ser485-phosphorylated AMPKα (pAMPKα), total AMPKα, Ser181-phosphorylated AMPKβ (pAMPKβ) and total AMPKβ. Whole-cell lysates from the livers of mice infected with adenovirus expressing short hairpin RNA targeted for LacZ , Gys2 or Pygl (Ad-LacZ-i, Ad-Gys2-i or Ad-Pygl-i). ( g ) Quantified results of the data shown in ( f ), shown as the ratio of pAMPKα to total AMPKα and pAMPKβ to total AMPKβ. ( n =3–4). All mice are analysed on 24-h fasting condition. * P <0.05 versus Ad-LacZ-i sham group (by Tukey’s post-hoc test). NS, not significant. Error bars, s.e.m. Full size image The results of this paper reveal that glycogen shortage in the liver triggers the liver–brain–adipose neural axis, promoting fatty acid and glycerol release from white adipose tissue as a response to fasting ( Supplementary Fig. S1 ). The presence of the liver–brain–adipose axis for the regulation of lipolysis in adipose tissue was first described by Katagiri et al . [6] They found that adenovirus-mediated expression of peroxisome proliferator-activated receptor γ2 in the liver induces acute hepatic steatosis, while markedly decreasing peripheral adiposity through afferent vagal signals originating in the liver, and that this neural pathway functions to protect against metabolic perturbation induced by pathologically excessive energy storage. By contrast to their finding, we have found that this neural axis has a physiological role and mediates the fasting signal from the liver to the adipose tissue under non-pathological conditions. Moreover, we have clarified that glycogen shortage in the liver triggers the neural axis during fasting. The liver is widely known to respond to a fasting state by activating various pathways, such as cAMP-activated kinase [7] , AMPK [8] , peroxisome proliferator-activated receptor α [9] and glucocorticoid receptor signalling [10] . However, the known upstream triggers of these pathways are all external signals derived outside the liver, such as changes in the levels of blood glucose, fatty acids, insulin, glucagon, epinephrine, glucocorticoids and so on. By contrast, we have shown that the neural axis is driven by an internal signal reflecting glycogen shortage in the liver. Although the question ‘What is the molecular identity of the glycogen sensor?’ remains unanswered, it is clearly demonstrated that liver itself senses glycogen shortage during fasting independently of changes in blood glucose or metabolic hormone levels. As a candidate glycogen sensor, it has been reported that the AMPKβ subunit binds to and is inhibited by glycogen in muscle [11] . However, our data from glycogen phosphorylase knockdown experiments ( Fig. 4f,g ) indicate that the blockade of glycogenolysis and the resultant higher glycogen levels suppresses the lipolytic activity through the liver–brain–adipose axis despite the activation of AMPK, suggesting that AMPK is not involved in this regulation. Consistent with this finding, AMPK is also reported to be hyperactivated in subjects with McArdle disease, who are unable to mobilize glycogen because of an inherited defect in glycogen phosphorylase, despite the presence of high glycogen levels [12] . Therefore, in our experimental model, AMPK was not thought to be the primary glycogen sensor in sensing the glycogen shortage and triggering the neural axis. It has been reported that glucocorticoid signals are also mediated by afferent vagal nerve pathway to control systemic insulin sensitivity and blood pressure [2] . Although we focused on adipose tissue as the effecter of the neurocircuitry in the present study, the liver-derived fasting signal transmitted through the vagal nerve might possibly have wider effects on the regulation of systemic energy metabolism. Further work is required to understand the overall system triggered by hepatic vagal nerve signals. In conclusion, our results demonstrated that the hepatic sensing of glycogen shortage activates a liver–brain–adipose neural axis to ensure energy availability by shifting the energy source from carbohydrates to fat. Materials Capsaicin were purchased from Wako Chemical (Tokyo, Japan). Guanethidine hemisulfate was purchased from Fluorochem (Derbyshire, UK). Anti-HSL, anti-phospho-HSL (ser 563), anti-ATGL, anti- phospho CRE-binding protein, anti- glycogen synthase, anti-AMPKα, anti- phospho AMPKα (Thr172), anti-AMPKβ1/2 and anti-phospho AMPKβ1 (Ser108) antibodies (rabbit polyclonal) were purchased from Cell Signaling Technology. Anti-PYGL (goat polyclonal) antibody was purchased from Santa Cruz Biotechnology. Animals Six to seven-week-old ICR mice were purchased from CLEA (Tokyo, Japan). All animals were maintained in a temperature-controlled environment with a 12 h-light/dark cycle and were given free access to standard laboratory diet and water. Mice were killed in the early light phase in a fasted or nonfasted ( ad libitum ) state. All animals studied were anaesthetised and euthanized according to protocol approved by the Tokyo University Animal Care and Use Committee. All experiments were repeated at least twice. Dissection of hepatic branch of the vagus Fourteen days before adenovirus administration, 7-week-old male mice were subjected to a selective HVx or to a sham operation (Sham). A laparotomy incision was made on the ventral midline and the abdominal muscle wall was opened with a second incision. The gastrohepatic ligament was severed using fine forceps, and the stomach was gently retracted, revealing the descending ventral oesophagus and the ventral subdiaphragmatic vagal trunk. The hepatic branch of this vagal trunk was then transected using fine forceps. Selective blockade of hepatic vagal afferent nerve For perivagal application of capsaicin, the hepatic branch of the vagal trunk was exposed as described above, then loosely tied with a cotton string immersed with or without capsaicin (Sigma Chemical) dissolved in olive oil (17%wt/vol) according to the modified Uno et al . [6] method. The cotton string was removed 30 min later and the abdominal incision was closed. Sympathetic nerve blockade For sympathetic nerve blockade experiments, Guanethidine (Fluorochem, Derbyshire, UK) was administered to 7-week-old male mice by a single i.p. injection (100 mg kg −1 ) 40 h before kill [4] . Preparation and transduction of recombinant adenoviruses The fragment containing CRE with SV40 promoter linked to luciferase reporter gene was inserted into the Gateway entry vector pENTR4 (Invitrogen) and adenoviral constructs were generated by homologous recombination between the entry vector and the pAd promoterless vector (Invitrogen). The sequence of CRE was as follows: 5′-CAGCCTGACGTCAGAGGCCTGACGTCAGAGAGCCTGACGTCAGAGAGCCTGACGTCAGA-3′. For adenovirus overexpressing Gys2 gene, cDNA encoding mouse Gys2 was PCR-amplified using primers 5′-GGTACCGCCACCATGCTCAGAGGCCGCTCC-3′ and 5′-CTCGAGATCATTTCGTTTGAGCTCAGTCAGTTC-3′ and subcloned into pENTR4 and then adenoviral constructs were generated by homologous recombination between the entry vector and the pAd/CMV/V5-DEST vector (Invitrogen). Adenoviruses encoding shRNA targeting LacZ , Gys2 and Pygl genes (LacZ-i, Gys2-i and Pygl-i, respectively) were constructed by cloning synthetic DNA into pENTR/U6 entry vector followed by homologous recombination with the pAd promoterless vector (Invitrogen). The target sequences are as follows: 5′-GCTAACGACATGCTCATAT-3′ for Gys2 and 5′-GGATAGTTATAATTGGTGG-3′ for Pygl . Recombinant adenoviruses were propagated in HEK293 cells and purified by CsCl gradient centrifugation as described previously [13] . Adenoviruses were injected intravenously into mice at the following doses: for expression of GFP , LacZ and Gys2 , 5 × 10 8 plaque-forming units (p.f.u. ); for LacZ-i, Gys2-i and Pygl-i, 7.5 × 10 8 p.f.u. In vivo imaging of luciferase activity In vivo imaging was performed as described previously [14] . Briefly, 1 × 10 8 p.f.u. of Ad-CRE-luc were delivered to epididymal fat in mice by micro syringe injection (Hamilton, Illinois, USA). Three to six days after the adenovirus transduction, 3.0 mg of D -luciferin potassium salt (Wako Chemical) was injected into mice and the luminescence in the adipose tissue was captured using an IVIS Imaging System (Xenogen) 15 min after the luciferin injection. Relative photon emission over the epididymal fat region was quantified using LivingImage software (Xenogen). RNA isolation and Northern blotting Total RNA preparation and blot hybridization with cDNA probes were performed as previously described [15] , [16] . Briefly, total RNA was isolated with Trizol reagent (Invitrogen), and 10 μg RNA samples equally pooled from mice of each group were run on a 1% agarose gel containing formaldehyde and transferred to a nylon membrane. The cDNA probes used for hybridization are listed in Supplementary Table S2 . The probes were labelled with [α-32P]dCTP using Megaprime DNA Labelling System kit (Amersham Biosciences). The membranes were hybridized with the radiolabeled probe in Rapid-hyb Buffer (Amersham Biosciences) at 65 °C, and washed three times in 0.1 × SSC, 0.1% SDS at 65 °C. Blots were exposed to BAS imaging plate for the BAS2000 BIO Imaging Analyser (Fuji Photo Film). Quantitative reverse transcription PCR Two micrograms of total RNA was reverse-transcribed using the High Capacity cDNA reverse transcription kit (Applied Biosystems). qRT–PCR was performed using SYBR Green Dye (Roche Applied Science) on a LightCycler480II (Roche Applied Science). The primer sets used for qRT–PCR are listed in Supplementary Table S3 . Metabolic measurements Levels of glucose, insulin, free fatty acids, glycerol and β-hydroxybutyrate in plasma and glycogen in the liver were measured as previously described [5] , [15] . Glucagon and leptin were measured in plasma using a Bio-Plex Panel (Bio-Rad) according to the manufacturer’s instructions. FGF21 in plasma was measured by FGF21 ELISA kit (R&D system, Minneapolis, USA). Immunoblotting Immunoblotting was performed as described previously [14] . Briefly, whole-cell lysates or tissue extracts were fractionated by SDS–PAGE and transferred to a polyvinylidene difluoride membrane using a transfer apparatus according to the manufacturer’s protocols (Bio-Rad). After blocking with 5% nonfat milk in TBS-T (10 mM Tris at pH 8.0, 150 mM NaCl, 0.5% Tween 20) for 30 min, the membrane was incubated with each primary antibody at 4 °C for 12 h. Membranes were washed three times for 10 min and incubated with a 1:2,000 dilution of horseradish peroxidase-conjugated second antibody for 1 h. The primary antibodies used for immunoblotting are listed in Supplementary Table S4 . Signals were detected using the ECL western blotting Detection System kit (Amersham Biosciences) and exposed to Kodak XAR-5 film and/or analysed using LAS-3000 imager (Fujifilm). DEXA analysis PIXImus2 DEXA (GE Medical Systems, LUNAR) was used to measure weight and per cent of lean body tissue and fat mass. Statistical differences between groups were analysed by ANOVA analysis of variance. Metabolic cage analysis After a 1-day acclimation period, oxygen and bicarbonate expired by 7-week-old male mice were measured every 7 min for 25 h by a calorimetric system (Alco System model, Chiba, Japan). Fat utilization and energy consumption were calculated by followed formula; fat utilization=1.67 × (VO 2 −VCO 2 ) (mg min −1 ), energy consumption=3.816 × VO 2 +1.231 × VCO 2 (cal min −1 ). Histological analysis White adipose tissue was removed and fixed with 10% formalin and embedded in paraffin. Tissue sections were stained with hematoxylin eosin. Total adipocyte areas were traced manually and quantified with the NIH image program. Statistical analyses Data are expressed as means±s.e.m. Differences between two groups were assessed using the unpaired two-tailed Student’s t -test unless otherwise noted. Data sets involving more than two groups were assessed by Tukey’s post-hoc test. The differences were considered to be significant if P <0.05. How to cite this article: Izumida, Y. et al . Glycogen shortage during fasting triggers liver–brain–adipose neurocircuitry to facilitate fat utilization. Nat. Commun. 4:2316 doi: 10.1038/ncomms3316 (2013).